Primary tumours modulate innate immune signalling to create pre-metastatic vascular hyperpermeability foci In mouse models of lung metastasis, before the appearance of significant metastases, localized changes in vascular permeability have been observed, which appear to set the stage for tumour growth. However, it is unclear whether this is also true in human patients. Here, we show that MD-2, a coreceptor for Toll-like receptor 4 that has a key role in the innate immune response, triggers the formation of regions of hyperpermeability in mice by upregulating C-C chemokine receptor type 2 (CCR2) expression. The CCR2–CCL2 system induces the abundant secretion of permeability factors such as serum amyloid A3 and S100A8. Disruption of MD-2 or CCR2 abrogates the formation of hyperpermeable regions, resulting in reduced tumour cell homing. Furthermore, fibrinogen, which is processed during permeability-mediated coagulation, is also localized in areas of elevated CCR2 expression in tumour-bearing human lungs. Our findings raise the possibility that CCR2 upregulation might represent a marker for regions of increased susceptibility to metastatic homing in lung cancer. Distant metastasis is a major cause of cancer mortality. During metastasis, cancer cells intravasate from the primary tumour, migrate to a secondary site via the blood vessels, extravasate into the surrounding tissue and form metastatic nodules [1] , [2] , [3] . In addition, some tumour cells initially reside in secondary organs in a dormant state, during which tumour expansion is blocked due to an inability to recruit new and functional blood vessels [4] . It is important to predict metastatic sites and detect dormant tumours that are at high risk of metastatic growth to improve the treatment of cancer. In the metastatic process, the ‘pre-metastatic phase’ has been recognized as a period during which organs acquire the character of hospitable soil for tumour cells before their arrival, and this process is facilitated by the distant primary tumour [5] , [6] . Several mechanisms have been suggested to be responsible for the creation of a pre-metastatic environment in the lungs, and many primary tumour-related factors such as cytokines, chemokines, amine oxidases and exosomes have been suggested to modify the lungs in order to facilitate the development of homing sites for circulating tumour cells [7] , [8] , [9] , [10] , [11] , [12] , [13] , [14] , [15] , [16] . In experimental metastasis models, pre-metastatic events, including bone marrow-derived cell (BMDC) mobilization and the activation of inflammatory pathways, have been found to affect the entire lung [7] , [8] , [9] , [10] , [11] , [12] , [13] , [14] , [15] , [16] . Although all pulmonary vessels seem to be exposed to these factors, spontaneous metastases often present an oligometastatic or solitary pattern in humans and mice [17] , [18] . In fact, we demonstrated that the above-mentioned vascular hyperpermeability regions contribute to subsequent tumour cell homing in lung vessels [19] and hypothesized that these regions are established through the induction of endothelial cell-dependent permeability via the upregulation of growth factor or chemokine receptors. Here, we demonstrate that innate immune signalling through Toll-like receptor 4 (TLR4) and its coreceptor MD-2 promotes the formation of regions of enhanced vascular permeability in tumour-bearing mouse lungs, through upregulation of chemokine signalling. CCL2-CCR2 enhances pre-metastatic vascular permeability To investigate the factors that affect the generation of vascular hyperpermeability regions in the pre-metastatic phase, we screened tumour-bearing mouse lungs for receptors that did not contain spontaneous metastases but might be able to respond to permeability factors from distant primary tumours. First, we found receptors whose expression was upregulated in Lewis lung carcinoma (LLC)-bearing mouse lungs compared with non-tumour-bearing mouse lungs using gene array analysis ( Supplementary Fig. S1a ). Then, we compared the gene expression levels of these receptors between hyperpermeable (H) and poorly permeable regions (L) in the tumour-bearing mouse lungs (permeability was determined by assessing the leakage of Evans blue (EB)) ( Fig. 1a ). Macroscopically, the hyperpermeable regions accounted for 5–10% of the surface area of the tumour-bearing lungs, and we collected dissected lung tissue from the hyperpermeable and poorly permeable regions of these lungs. Of the examined genes, C-C chemokine receptor type 2 ( CCR2 ) showed the largest increase in its expression (13.1-fold) between the hyperpermeable regions of the tumour-bearing lungs and the poorly permeable regions of the non-tumour-bearing mouse lungs, where EB leakage was very low, as was also the case in the poorly permeable regions in the tumour-bearing mice ( Supplementary Fig. S1b ). As a previous study found that metastatic cancer cells preferentially homed to the hyperpermeable foci in LLC- or E0771-mammary carcinoma-bearing-lungs [19] , we examined whether CCR2 expression was upregulated in the hyperpermeable regions induced by E0771-tumour cells in syngeneic C57BL/6 mice. In addition, we also used tumour-conditioned media (TCM) to stimulate the production of these regions in order to eliminate the possibility of micrometastasis-mediated vascular hyperpermeability in the pre-metastatic lungs. To examine the relationship between EB-leakage sites and the localization of CCR2 and its ligand CCL2, we carried out immunohistochemical analyses ( Supplementary Figs S2,S3 ), which confirmed that the hyperpermeable foci overlapped with areas of upregulated CCL2-CCR2 expression in E0771-mammary fat pad (mfp)-bearing ( Fig. 1b ), E0771-tumour-conditioned medium (ETCM)-stimulated ( Fig. 1b ), and LLC-bearing (data not shown) mouse lungs. Next, we characterized the cell types of the CCR2-positive cells in the hyperpermeable regions of the tumour-bearing mouse lungs. We first examined the expression of cell markers such as MECA32, CD45, CC10 and Lyve-1, which are markers of endothelial cells, pan-leukocytes, lung epithelial cells and lymphatic cells, respectively, in the CCR2-positive cells in the regions of high EB leakage (EB-high). Among them, the CCR2-positive cells mainly expressed CD45 (~65%) or MECA32 (~35%), as shown in Supplementary Figs. S2b and S4 . Most lymphatic vessels did not express CCR2, but ~1.5% of the Lyve-1-positive lymphatic cells clearly expressed CCR2 ( Supplementary Fig. S5 ). 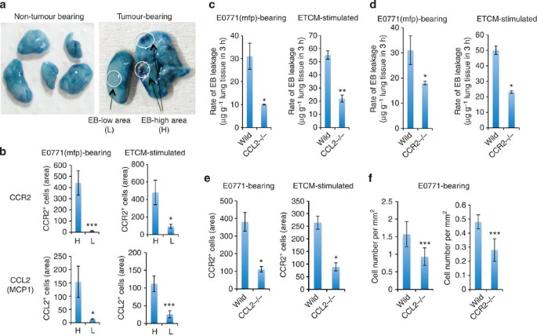Figure 1: The CCL2–CCR2 system generates discrete hyperpermeable regions in pre-metastatic mouse lungs. (a) Distinct macroscopic regions of EB leakage were observed in the lungs of the tumour-bearing mice (EB-high: hyperpermeable area, EB-low: poorly permeable area). (b) Upregulation of CCL2 and CCR2 expression in the hyperpermeable areas of E0771(mfp)-bearing or ETCM-stimulated mouse lungs. Mfp, mammary fat pad; ETCM, E0771-cultured conditioned media. (n=5) (c,d) Reduced EB leakage was observed in the E0771-bearing or ETCM-stimulated CCL2−/− (c) or CCR2−/− (d) mouse lungs. (e) Suppression of CCR2 expression in tumour-stimulated CCL2−/− mouse lungs. (f) Reduced tumour cell accumulation was observed in the E0771-bearing CCL2−/− and CCR2−/− mouse lungs.n=4 (c–f). Error bars indicate the mean±s.e.m., andP-values are relative to the wild-type (c–f). Student’st-test, *P<0.05, **P<0.01, ***P<0.005. Figure 1: The CCL2–CCR2 system generates discrete hyperpermeable regions in pre-metastatic mouse lungs. ( a ) Distinct macroscopic regions of EB leakage were observed in the lungs of the tumour-bearing mice (EB-high: hyperpermeable area, EB-low: poorly permeable area). ( b ) Upregulation of CCL2 and CCR2 expression in the hyperpermeable areas of E0771(mfp)-bearing or ETCM-stimulated mouse lungs. Mfp, mammary fat pad; ETCM, E0771-cultured conditioned media. ( n =5) ( c , d ) Reduced EB leakage was observed in the E0771-bearing or ETCM-stimulated CCL2−/− ( c ) or CCR2−/− ( d ) mouse lungs. ( e ) Suppression of CCR2 expression in tumour-stimulated CCL2−/− mouse lungs. ( f ) Reduced tumour cell accumulation was observed in the E0771-bearing CCL2−/− and CCR2−/− mouse lungs. n =4 ( c – f ). Error bars indicate the mean±s.e.m., and P -values are relative to the wild-type ( c – f ). Student’s t -test, * P <0.05, ** P <0.01, *** P <0.005. Full size image In order to examine the functional role of this system, we used CCL2 and CCR2 knockout mice. We first confirmed that lung vascular permeability did not differ among the wild-type, CCL2−/− and CCR2 −/− mice without tumours (data not shown). No focal vascular hyperpermeability regions were observed in the E0771-bearing or ETCM-stimulated CCL2- or CCR2-depleted mouse lungs, resulting in a reduction in total EB leakage in these mice compared with the wild-type mice ( Fig. 1c ). As ligands sometimes affect the expression of their receptors [20] , we examined the levels of CCR2 protein in tumour-bearing- or TCM-stimulated-CCL2−/− mouse lungs. As a result, we found that the changes in CCR2 expression induced by the primary tumours were dependent on CCL2 ( Fig. 1e ). Finally, we examined whether the CCL2–CCR2 system was involved in the accumulation of circulating tumour cells with metastatic potential at hyperpermeable regions in the tumour-bearing mice. To study the metastatic phase in these mice, we intravenously injected fluorescence-labelled tumour cells into tumour-bearing mice to mimic spontaneous metastasis (see ‘Experimental metastatic model’ in Methods and Supplementary Fig. S6 ). Owing to the lack of hyperpermeable foci in the tumour-bearing CCL2 or CCR2 knockout mice, tumour cell homing was suppressed in these mice ( Fig. 1f ). Thus, CCL2 and CCR2 might contribute to the formation of spontaneous macroscopic metastases because lung metastases derived from subcutaneous 3LL tumours, a highly metastatic line, were also suppressed in both types of knockout mice ( Supplementary Fig. S7 ). Moreover, after tumour cell accumulation in the lungs, the hyperpermeable regions supported tumour cell survival and proliferation, as evidenced by the fact that fewer TUNEL-positive and more Ki67-positive tumour cells were seen in the hyperpermeable regions than in the poorly permeable regions ( Supplementary Figs S8,S9 ). CCL2 and inflammatory mediators stimulate lung permeability As CCL2-CCR2 signalling regulates inflammatory monocytes [21] and the expression levels of inflammatory mediators such as S100A8, S100A9 and serum amyloid A3 (SAA3) are upregulated in pre-metastatic lungs [8] , [9] , we examined the expression of these molecules in the focal hyperpermeable regions in the tumour-bearing mouse lungs. The mRNA and protein levels of S100A8, S100A9 and SAA3 were increased in the highly permeable regions ( Fig. 2a , Supplementary Figs S10,S11 ), and a marked induction of SAA3 protein expression was observed in the endothelial cells in the EB-high areas of the E0771-bearing mice ( Supplementary Fig. S12 ). Furthermore, the induction of SAA3 protein expression was clearly regulated by CCL2 in the E0771-bearing and ETCM-stimulated mice ( Fig. 2b ). 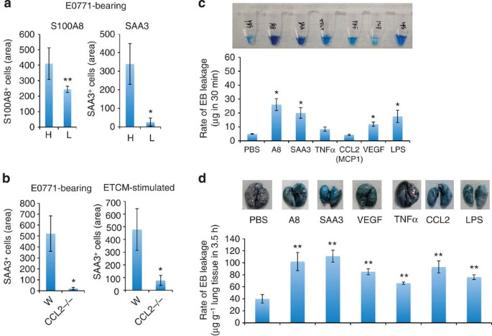Figure 2: Inflammatory factors strongly induce the development of hyperpermeable regions in wild-type mouse lungs. (a) S100A8 and SAA3 expression were upregulated in the hyperpermeable (H) regions, but not the poorly permeable (L) regions of the E0771-bearing mouse lungs (n=6). (b) Inhibition of SAA3 expression in E0771-bearing or ETCM-stimulated CCL2−/− mouse lungs (n=4). (c) S100A8- (A8) or SAA3-induced peritoneal leakage of EB (n=6). Representative peritoneal EB leakage is shown in the upper panel. (d) CCL2, S100A8 and SAA3-stimulated EB leakage in mouse lungs (n=6). Student’st-test, *P<0.05, **P<0.01. Figure 2: Inflammatory factors strongly induce the development of hyperpermeable regions in wild-type mouse lungs. ( a ) S100A8 and SAA3 expression were upregulated in the hyperpermeable (H) regions, but not the poorly permeable (L) regions of the E0771-bearing mouse lungs ( n =6). ( b ) Inhibition of SAA3 expression in E0771-bearing or ETCM-stimulated CCL2−/− mouse lungs ( n =4). ( c ) S100A8- (A8) or SAA3-induced peritoneal leakage of EB ( n =6). Representative peritoneal EB leakage is shown in the upper panel. ( d ) CCL2, S100A8 and SAA3-stimulated EB leakage in mouse lungs ( n =6). Student’s t -test, * P <0.05, ** P <0.01. Full size image To examine whether inflammatory factors directly or indirectly contribute to vascular hyperpermeability in vivo , we carried out traditional permeability assays such as skin and peritoneal leakage assays involving the intradermal and intraperitoneal injection of various factors followed by intravenous EB injection. To see whether the examined factors had the ability to directly stimulate vascular permeability, we first carried out a Miles assay using mouse skin to trace the time course of the development of vascular permeability. As a result, we found that mouse S100A8 and SAA3, but not CCL2, produced immediate and strong permeability responses at 5–15 min after their injection ( Supplementary Fig. S13 ). We obtained similar results for S100A8 and SAA3 in a peritoneal permeability assay. In the latter assay, S100A8- and SAA3-induced vascular hyperpermeability to a similar extent to the positive controls, vascular endothelial growth factor (VEGF) and lipopolysaccharide (LPS) ( Fig. 2c ). In the lungs, the hyperpermeability was strongest in the foci after 3–5 h. Interestingly, CCL2 stimulated lung permeability to the same extent as SAA3 and S100A8 ( Fig. 2d ). Granulocyte colony-stimulating factor, whose receptor was also a candidate molecule ( Supplementary Fig. S1 ), did not induce marked focal lung hyperpermeability ( Supplementary Fig. S14 ). Furthermore, we performed an in vivo experiment to investigate whether CCL2 was involved in the focal lung hyperpermeability induced by the TCM. As shown in Supplementary Fig. S15 , the administration of an anti-CCL2 antibody reduced ETCM-mediated focal lung hyperpermeability. Upregulation of CCR2 and S100A8/A9 in lungs from cancer patients To evaluate whether CCR2 expression is upregulated in regions of increased vascular permeability in tumour-bearing human lungs, we tried to detect hyperpermeable areas by searching for regions in which fibrinogen expression had been induced. Fibrinogen is a reliable biomarker of inflammation, and its degradation products have been found to be associated with microvascular leakage [22] , [23] . In the present study, we found that fibrinogen expression was increased in the hyperpermeable regions of the tumour-bearing mouse lungs compared with the poorly permeable regions and that its upregulation occurred in the same regions as the upregulation of CCR2 ( Fig. 3a ). An experiment in which we induced acute vascular permeability via TCM stimulation produced similar results ( Fig. 3a ). To determine the optimal condition of the analysis in human samples, we first tested the relationships among vascular hyperpermeability, fibrinogen expression and CCR2 expression in tumour-bearing mouse lungs in areas with various diameters (50–400 μm), and found significant differences between the hyperpermeable and poorly permeable regions, regardless of the diameter of the area (data not shown). Thus, we applied the largest area (400 μm) for the subsequent analysis of human samples because vascular hyperpermeability usually results in the formation of macroscopic EB leakage foci. 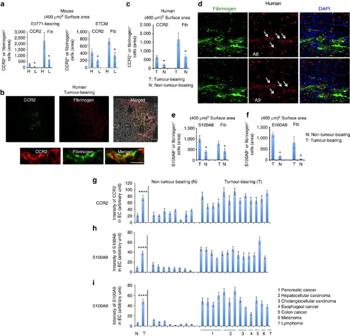Figure 3: Increased CCR2 expression is observed in regions of increased fibrinogen expression in tumour-bearing human lungs. (a) In E0771-bearing or TCM-stimulated mouse lungs, CCR2 and fibrinogen expression were upregulated in the hyperpermeable (H) regions compared with the poorly permeable (L) regions (n=5). (b) Representative staining of CCR2 and fibrinogen in tumour-bearing human lungs. Co-localization of CCR2 and fibrinogen in a relatively large region (upper, scale bar, 1 mm) and a magnified image (lower, scale bar, 50 μm). (c) The lungs of the tumour-bearing patients (n=13) displayed increased CCR2 and fibrinogen expression compared with those of the non-tumour-bearing patients (n=8). (d) Representative staining of the co-localization of S100A8, S100A9 and fibrinogen in tumour-bearing human lungs. (e,f) Increased S100A8/A9 and fibrinogen expression were observed in the lungs of the tumour-bearing patients. (g–i) Summary of the expression levels of CCR2, S100A8 and S100A9 in endothelial cells. The mean expression intensities of each molecule in lung tissue from patients with no tumours and patients with various tumours are shown in the left columns. Student’st-test, *P<0.05, ****P<0.001. Figure 3: Increased CCR2 expression is observed in regions of increased fibrinogen expression in tumour-bearing human lungs. ( a ) In E0771-bearing or TCM-stimulated mouse lungs, CCR2 and fibrinogen expression were upregulated in the hyperpermeable (H) regions compared with the poorly permeable (L) regions ( n =5). ( b ) Representative staining of CCR2 and fibrinogen in tumour-bearing human lungs. Co-localization of CCR2 and fibrinogen in a relatively large region (upper, scale bar, 1 mm) and a magnified image (lower, scale bar, 50 μm). ( c ) The lungs of the tumour-bearing patients ( n =13) displayed increased CCR2 and fibrinogen expression compared with those of the non-tumour-bearing patients ( n =8). ( d ) Representative staining of the co-localization of S100A8, S100A9 and fibrinogen in tumour-bearing human lungs. ( e , f ) Increased S100A8/A9 and fibrinogen expression were observed in the lungs of the tumour-bearing patients. ( g – i ) Summary of the expression levels of CCR2, S100A8 and S100A9 in endothelial cells. The mean expression intensities of each molecule in lung tissue from patients with no tumours and patients with various tumours are shown in the left columns. Student’s t -test, * P <0.05, **** P <0.001. Full size image To assess whether distant primary tumours stimulate the co-localized induction of fibrinogen and CCR2 expression in tumour-bearing human lungs, we examined the expression of both molecules in healthy lung regions from patients who carried tumours in their extra-pulmonary organs. At first, we microscopically examined the lung lobes to find healthy regions without tumour metastasis, atelectasis or inflammation. As a control, we detected relatively low levels of fibrinogen and CCR2 in lungs from patients without tumours ( Fig. 3c ). In contrast, the co-localization of upregulated fibrinogen and CCR2 expression was detected in the lungs of patients with tumours, such as pancreatic cancer, hepatocellular carcinoma and cholangiocellular carcinoma ( Fig. 3b ). It was reported that carcinoma patients displayed higher serum S100A8 and S100A9 proteins concentrations than adenoma patients [24] , and we also confirmed slight but appreciable increases in the serum S100A9 levels of patients with various tumours (data not shown). We also observed the co-localization of increased S100A8 or S100A9 levels with upregulated fibrinogen expression in the lungs of tumour-bearing patients ( Fig. 3d–f ). Next, we examined the correlation between CCR2 and S100A8/A9 expression based on our mouse data. Again, the tumour-bearing lung endothelial cells exhibited significantly increased CCR2 and S100A8/A9 expression levels compared with the non-tumour-bearing lungs ( Fig. 3g–i , Supplementary Fig. S16 ). The CCL2-S100A8/A9-SAA3 cascade requires MD-2 In the lungs, both extrinsic and intrinsic factors induce vascular permeability. To examine whether these permeability-inducing factors also stimulate S100A8 and/or SAA3 expression, we applied them to lung organ cultures. Among them, CCL2 stimulated S100A8 and S100A9 expression more prominently than VEGF ( Fig. 4a ). Furthermore, CCL2 stimulated an autocrine cascade as it upregulated the expression of CCL2 and CCR2 ( Fig. 4a ). On the contrary, LPS, but not VEGF or CCL2, markedly induced tumour necrosis factor (TNF)-α expression ( Fig. 4a ). We detected similar patterns at the protein level ( Fig. 4b ). 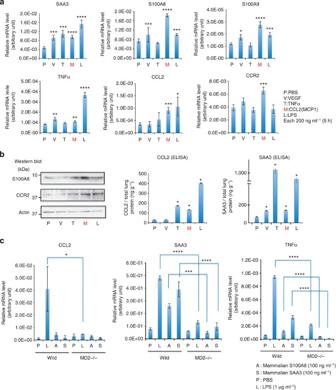Figure 4: The CCL2–CCR2 system triggers the expression of S100A8/A9-SAA3 via MD-2 in lung organ cultures. (a) CCL2 stimulatedSAA3, S100A8, S100A9, CCL2andCCR2expression in wild-type mouse lungs in organ cultures. mRNA levels were measured by quantitative-PCR at 5 h after treatment with PBS, VEGF, TNFα, CCL2 or LPS and normalized to that of β-actin (n=3). (b) CCL2 upregulated SAA3, S100A8, CCL2 and CCR2 protein expression, as detected by western blotting and enzyme-linked immunosorbent assay (ELISA) in lung organ cultures. (c) Mouse S100A8 and SAA3 derived from mammalian cells stimulatedSAA3andTNFα expression via MD-2 in lung organ cultures. mRNA levels were measured by quantitative-PCR at 6 h after the application of PBS, LPS, S100A8 or SAA3 and were normalized to that of β-actin (n=3). Student’st-test, *P<0.05, **P<0.01, ***P<0.005, ****P<0.001. Figure 4: The CCL2–CCR2 system triggers the expression of S100A8/A9-SAA3 via MD-2 in lung organ cultures. ( a ) CCL2 stimulated SAA3, S100A8, S100A9, CCL2 and CCR2 expression in wild-type mouse lungs in organ cultures. mRNA levels were measured by quantitative-PCR at 5 h after treatment with PBS, VEGF, TNFα, CCL2 or LPS and normalized to that of β-actin ( n =3). ( b ) CCL2 upregulated SAA3, S100A8, CCL2 and CCR2 protein expression, as detected by western blotting and enzyme-linked immunosorbent assay (ELISA) in lung organ cultures. ( c ) Mouse S100A8 and SAA3 derived from mammalian cells stimulated SAA3 and TNF α expression via MD-2 in lung organ cultures. mRNA levels were measured by quantitative-PCR at 6 h after the application of PBS, LPS, S100A8 or SAA3 and were normalized to that of β-actin ( n =3). Student’s t -test, * P <0.05, ** P <0.01, *** P <0.005, **** P <0.001. Full size image Toll-like receptors (TLR), which recognize both extrinsic and intrinsic ligands, have key roles in the activation of inflammation and the innate immune response [25] , [26] , [27] . Among them, TLR4 is the receptor for intrinsic factors such as S100A8 and SAA3, as well as the extrinsic ligand LPS. Recently, the crystallographic structure of TLR4–MD-2–LPS complex has been elucidated [28] , [29] . It was demonstrated that the structural changes in MD-2 that occur after its binding to LPS are necessary for TLR4 dimer formation and the subsequent initiation of downstream signalling. Next, we investigated the MD-2 dependency of the CCL2-S100A8/A9-SAA3 cascade in lung organ cultures. Neither S100A8 nor SAA3 significantly induced CCL2 expression compared with that induced by LPS via MD-2 ( Fig. 4c ). On the other hand, both proteins stimulated SAA3 and TNF- α expression in an MD-2-dependent manner ( Fig. 4c ). Endothelial and leukocyte MD-2 mediate lung permeability We next examined whether the vascular permeability induced by SAA3 was dependent on signalling through MD-2 in vivo . As shown in Fig. 5a and Supplementary Fig. S17 , the peritoneal leakage induced by SAA3 was reduced in MD-2−/− mice. The discrete vascular hyperpermeability regions produced in response to primary E0771 tumours were almost absent from the MD-2 knockout mice ( Fig. 5b , upper), resulting in the suppression of lung leakage ( Fig. 5b , lower). A similar result was seen in E0771-bearing TLR4−/− mice (data not shown). In the metastasis assay, the injected tumour cells tended to accumulate in the focal hyperpermeable regions in the tumour-bearing wild-type mice. In accordance with the amelioration of vascular hyperpermeability in the E0771-bearing MD-2−/− mouse lungs, the accumulation of circulating tumour cells was diminished in the E0771- and LLC-bearing MD-2−/− mice ( Fig. 5c ). Spontaneous metastasis to the lungs was also reduced in the MD-2-depleted mice compared with the wild-type mice although the sizes of the primary E0771 and 3LL tumours did not differ significantly between the two genotypes ( Fig. 5d and Supplementary Fig. S18 ). 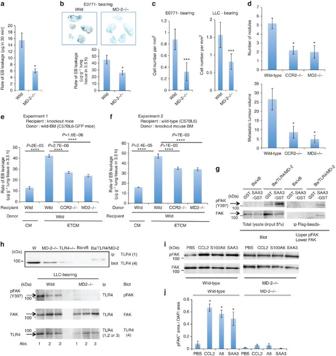Figure 5: MD-2 regulates inflammatory hyperpermeability by binding to TLR4-pFAK in the pre-metastatic phase. (a) Blockade of SAA3-mediated peritoneal permeability in MD-2−/− mice. (b) Inhibition of the formation of distinct regions of vascular hyperpermeability in E0771-bearing MD-2−/− mouse lungs (n=4). (c) Reduced tumour cell accumulation was observed in the E0771-bearing or LLC-bearing MD-2−/− mouse lungs (n=4). (d) Suppression of E0771 spontaneous metastases in MD-2−/− mice (n=5). (e,f) Suppression of TCM-mediated hyperpermeability in mice subjected to BMT in which CCR2 or MD-2 was knocked down in the donor BM or recipient cells. (g,h) Western blot analyses. Binding of TLR4/MD-2 to pFAK in SAA3-stimulated TLR4/MD-2-overexpressing (Ba/TLR4/MD-2) cells (g). Ba/κB cells were used as a negative control for Ba/TLR4/MD-2. Characterization of the TLR4 antibody in lysates from wild-type, MD-2−/− or TLR4−/− mouse lungs, Ba/κB cells and Ba/TLR4/MD-2 cells (h, upper). No binding of TLR4 to pFAK was observed in the LLC-bearing MD-2−/− mouse lungs. The TLR4 antibodies (no. 1–4) are described in the Methods section. The faint band in the TLR4−/− lane is non-specific (h, upper). (i,j) Suppression of CCL2, S100A8 and SAA3-induced pFAK expression in endothelial cells derived from MD-2−/− mice. pFAK signals were detected by western blotting (i) and quantified immunohistochemically (j). Student’st-test, *P<0.05, ***P<0.005. Figure 5: MD-2 regulates inflammatory hyperpermeability by binding to TLR4-pFAK in the pre-metastatic phase. ( a ) Blockade of SAA3-mediated peritoneal permeability in MD-2−/− mice. ( b ) Inhibition of the formation of distinct regions of vascular hyperpermeability in E0771-bearing MD-2−/− mouse lungs ( n =4). ( c ) Reduced tumour cell accumulation was observed in the E0771-bearing or LLC-bearing MD-2−/− mouse lungs ( n =4). ( d ) Suppression of E0771 spontaneous metastases in MD-2−/− mice ( n =5). ( e , f ) Suppression of TCM-mediated hyperpermeability in mice subjected to BMT in which CCR2 or MD-2 was knocked down in the donor BM or recipient cells. ( g , h ) Western blot analyses. Binding of TLR4/MD-2 to pFAK in SAA3-stimulated TLR4/MD-2-overexpressing (Ba/TLR4/MD-2) cells ( g ). Ba/κB cells were used as a negative control for Ba/TLR4/MD-2. Characterization of the TLR4 antibody in lysates from wild-type, MD-2−/− or TLR4−/− mouse lungs, Ba/κB cells and Ba/TLR4/MD-2 cells ( h , upper). No binding of TLR4 to pFAK was observed in the LLC-bearing MD-2−/− mouse lungs. The TLR4 antibodies (no. 1–4) are described in the Methods section. The faint band in the TLR4−/− lane is non-specific ( h , upper). ( i , j ) Suppression of CCL2, S100A8 and SAA3-induced pFAK expression in endothelial cells derived from MD-2−/− mice. pFAK signals were detected by western blotting ( i ) and quantified immunohistochemically ( j ). Student’s t -test, * P <0.05, *** P <0.005. Full size image We next tried to assess the extent to which the CCR2-MD-2 in endothelial cells, lymphatic cells and CD45 + -leukocytes contributes to the vascular hyperpermeability observed in primary tumour-stimulated mouse lungs. To generate mice in which CCR2 was specifically depleted in the resident lung cells, including endothelial/lymphatic cells, or BMDCs, including CD45 + cells, we carried out reciprocal bone marrow transplantation (BMT). To suppress CCR2 expression in the BMDC and resident lung cells, we generated CCR2−/−(donor)/wild-type(recipient) and wild-type(donor)/CCR2−/−(recipient) mice, respectively. We also produced MD-2−/−(donor)/wild-type(recipient) and wild-type(donor)/MD-2−/−(recipient) mice for the same assay system to examine the downstream cascade initiated by CCR2. In the BMT CCR2−/− mice, TCM-stimulated vascular hyperpermeability was decreased by 38 and 51% in the CCR2−/−(donor)/wild-type(recipient) and wild-type(donor)/CCR2−/−(recipient) mice, respectively, compared with that observed in the wild-type(donor)/wild-type(recipient) mice ( Fig. 5e and Table 1 ). Furthermore, both types of MD-2−/− mice showed similar patterns to the CCR2−/− mice ( Fig. 5e and Table 1 ). These results suggest that the CCR2-MD-2 axis in endothelial/lymphatic cells and CD45 + -leukocytes contributes to the formation of hyperpermeability foci in the tumour-bearing state. Table 1 Permeability reduction rates in BMT mice. Full size table CCL2-S100A8-SAA3 induces permeable foci via TLR4-FAK We previously showed that the vascular hyperpermeability induced in response to primary tumours was suppressed by the blockade of endothelial focal adhesion kinase (FAK) [19] . Based on this result, we investigated whether TLR4/MD-2 signalling exhibited cross-talk with FAK. The administration of SAA3 or S100A8 induced the phosphorylation of FAK (pFAK) in TLR4/MD-2-overexpressing cells. Both mammalian-derived murine SAA3 and glutathione S-transferase (GST)-fused SAA3 protein in the presence of polymyxin B induced pFAK ( Supplementary Fig. S19 ). Importantly, the pFAK protein bound to the Flag-tagged TLR4/MD-2 complex in these cells within 30 min of SAA3 stimulation ( Fig. 5g ). The binding of TLR4 to pFAK was observed in the LLC-bearing wild-type but not the MD-2−/− mouse lungs ( Fig. 5h ). Next, we tried to search for CCL2-dependent signalling in lung endothelial cells. First, we collected CD31 + /CD102 + lung endothelial cells. The collected cells were confirmed by an another endothelial-specific marker VE-cadherin. As it has been reported that CCL2 stimulated p38-, Jak2- and PI3K-dependent cascades [30] , [31] , we examined whether these signalling cascades contribute to S100A8/A9 and SAA3 expression. The wild-type endothelial cells that were cultured with 0.4% TCM exhibited p38 and JAK2 phosphorylation after the application of CCL2 ( Supplementary Fig. S20 ). After treatment with inhibitors against p38, JAK2 or AKT; that is, SB203580, AG490 and Wortmannin, respectively, CCL2-mediated S100A8/A9 and SAA3 expression were blocked by SB203580 and AG490, respectively ( Supplementary Fig. S21 ). We also confirmed that the p38 and JAK2-dependent cascades upregulated SAA3 protein expression ( Supplementary Fig. S22 ). We then examined whether the above-mentioned inhibitors also blocked the pFAK signalling induced by CCL2. Both SB203580 and AG490 suppressed CCL2-mediated pFAK signalling in CD31 + /CD102 + lung endothelial cells ( Supplementary Figs S23,S24 ). We finally confirmed that CCL2-, S100A8- and SAA3-mediated pFAK signalling were inhibited in lung endothelial cells derived from MD-2−/− mice ( Fig. 5i ). These data indicate that MD-2 is a key molecule in the regulation of hyperpermeability foci via the TLR4-FAK cascade. The innate immune system regulates the balance between tumour progression and antitumour immunity. Recently, it has been reported that immune/inflammatory factors and cells have dual roles in tumour cells. If host-mediated antitumour immunity, such as that mediated by IL-10, IL-12 and IL-23, is stronger than tumour-mediated immunosuppressive activity, tumour cells are eliminated [32] . On the other hand, inflammatory mediators, including TNFα, IL-6 and IL-17, lead to the eradication of antitumour immunity and accelerated tumour progression. As for the TLR4-mediated immune system, it has also been reported to have a paradoxical role in tumour development. TLR4 signalling induces the production of IFN and cytokines with antitumour effects [33] . In contrast, the activation of TLR4 via the intraperitoneal injection of bacterial LPS stimulated the growth of lung metastases in a mouse model of transplanted metastatic cancers [33] , indicating that TNFα might enhance the growth of lung metastases as a major host-produced factor. From our data, host-derived factors belonging to the innate immune system facilitate metastasis via the TLR4/MD-2 system, which is established in the pre-metastatic phase. In a tumour-bearing state, which is similar to chronic inflammation, many primary tumour-derived factors, including CCL2, TNFα and VEGF, directly and indirectly stimulate CCR2 in potentially hyperpermeable areas, further inducing the secretion of SAA3 and S100A8, which increase vascular permeability via TLR4/MD-2. In addition, these factors might attract peripheral leukocytes and BMDC to focal hyperpermeability regions, which might in turn result in the infiltration of tumour cells into discrete hyperpermeable regions. It has been reported that the serum CCL2 protein levels of tumour-bearing patients were increased [34] and that the CCL2–CCR2 system is involved in offensive and defensive actions against inflammatory monocytes and neutrophils in lung metastases [35] , [36] . Lung metastasis sites attract both tumour cells and host defense cells. In addition, lungs from patients with distant primary tumours exhibited regions in which upregulated CCR2 expression and hyperpermeability/inflammation-related fibrinogen expression co-localized. The ability to predict and treat such regions might significantly contribute to the suppression of metastasis. Reagents The mouse VEGF, CCL2/monocyte chemotactic protein (MCP)-1, TNFα, anti-CCL2 Ab, anti-VEGF Ab, rabbit IgG, rat IgG, goat IgG and the enzyme-linked immunosorbent assay kit for CCL2 were purchased from R&D Systems. The EB, LPS ( E. coli LPS serotype 055:B5) and anti-Flag M2 agarose beads were from Sigma. The anti-CCR2 Ab (ab21667), anti-pFAK (Y397) Ab (ab4803) and anti-MD-2 Ab (ab73550) were from Abcam. The anti-CC10 Ab, anti-Lyve-1 Ab, and enzyme-linked immunosorbent assay kit for SAA3 were from Millipore. The anti-CCR2 Ab (sc-6228) and anti-VE-cadherin Ab were from Santa Cruz. The anti-Ki-67 Ab (clone SP6), in Situ Cell Death Detection kit and Cell Counting Kit-8 were obtained from Spring Bioscience, Roche and Dojindo, respectively. Animals CCR2−/− and CCL2−/− mice were purchased from The Jackson Laboratory. MD-2−/− mice were obtained from the RIKEN Bio Resource Center [37] . The TLR4−/− mice have been described previously [38] . The C57BL6 mice were purchased from CLEA and SLC. All animal procedures were performed according to the guidelines of the Animal Research Committee of Tokyo Women’s Medical University. Human samples All autopsy samples were analysed under approval by the Institutional Review Board of the Tokyo Women’s Medical University. Tumour cell lines and tumour-conditioned medium The E0771 breast cancer cell line was originally established by Dr Sirotnak (Memorial Sloan-Kettering Cancer Center, New York) and was kindly provided by Dr Mihich (Roswell Park Memorial Institute, Buffalo, NY) [39] . The 3LL cell line was provided by the National Cancer Institute. The C57BL/6 mouse-syngeneic LLC cell line and E0771 cells were maintained in Dulbecco’s modified Eagle’s medium (DMEM, ATCC) supplemented with 10% fetal bovine serum (FBS), 1,000 units ml −1 penicillin G sodium and 100 μg ml −1 streptomycin sulphate. To obtain TCM, the cell lines were incubated overnight in serum-free medium. Experimental metastatic model The period when the primary tumour was growing was considered to be the pre-metastatic phase, and the metastatic phase was defined as the period after the intravenous (i.v.) injection of the tumour cells into tumour-bearing mice. Syngeneic tumour grafts were generated via the subcutaneous (s.c.) or mammary fat pads (mfp) implantation of 5 × 10 6 LLC or E0771 cells into 8- to 10-week-old mice. We injected tumour cells into mice that possessed growing primary tumours of the same size. For the tumour cell homing assays, 2–10 × 10 4 rhodamine-labelled metastatic cells and fluorescent dye (PKH-26, Sigma) were infused into the mice via their tail veins. At 24 h after the cancer cell infusion, the lungs were perfused with phosphate-buffered saline (PBS) under physiological pressure to eliminate any circulating tumour cells and then excised. Four to six randomly selected lung tissue fragments (3 mm in diameter) were selected, and three 10-μM sections per fragment were examined using confocal microscopy. The labelled cancer cell counts were normalized to the total tissue surface area. Age- and sex-matched C57BL/6 mice were used as controls because the knockout mice were back-crossed on the C57BL/6 strain over ten generations. Spontaneous metastasis assay 3LL tumours were s.c. implanted into male C57BL/6 mice, and E0771 tumours were implanted into mammary fat pads (mfp) or s.c. implanted into female C57BL/6 mice ( n =5–6 mice). The primary tumours were resected when they reached a diameter of 13 mm (E0771), as tumours of this size were shown to reproducibly induce lung metastasis in pilot studies. Lung tissue was isolated from the mice at 2–4 weeks after the implantation (3LL) or removal of the primary tumour (E0771). Bone marrow transplantation C57BL/6 mice (8-week-old) were lethally irradiated by delivering a 9-Gy fraction to the whole body. The irradiated mice were rescued 24 h later by bone marrow transplants isolated from green fluorescent protein/C57BL/6 mice. Eight weeks after the BMT, we confirmed over 90–95% of the target BMDC had been replaced with green fluorescent protein-bone marrow cells using flow cytometry. After we had determined the optimal irradiation conditions for C57BL/6 mice, we carried out BMT using mice of different genotypes. Vascular permeability/leakage assays In the peritoneal vascular permeability assays, recombinant proteins (200 ng per 500 μl) were i.p. injected, followed by the i.v. injection of EB (200 μl of 20 mg ml −1 ). Assays of lung vascular permeability were performed once the tumours reached ~6–7 mm in diameter via the i.v. infusion of EB. In separate experiments, TCM or CM (media conditioned without tumour cells) was i.v. injected followed by EB. The CM was used as a control. The gene and protein expression levels in the EB-high and EB-low areas were measured using quantitative-PCR and immunohistochemistry. Quantification of EB leakage EB leakage was quantified at 30 min and 3–3.5 h after the EB infusion in the peritoneal and lung permeability assays, respectively, as described previously [19] . In brief, the pulmonary microvasculature was first flushed with PBS under physiological pressure. The lungs were then excised, rinsed in PBS and snap-frozen in liquid nitrogen. The frozen tissue was later homogenized in formamide/PBS and incubated at 60 °C for 16 h. To determine the EB concentration, we recorded the absorbance of the supernatant at 620 (A620) and 740 nm (A740). Tissue EB content (μg EB per g lung) was calculated by correcting the A620 value for the amount of haem pigment and comparing this value to a standard curve for EB in formamide/PBS. Isolation of endothelial cells We followed a previously described lung endothelial cell collection method [40] . In brief, minced newborn mouse lungs were digested with 1 mg ml −1 of collagenase, 1 mg ml −1 of dispase and DNase at 37 °C for 30 min. The lung cells were incubated with magnetic bead(Invitrogen)-conjugated anti-mouse CD31 antibody (R&D) and cultured on gelatin-coated plates for 3 days. After removing the cells that had bound to the beads, we further sorted them with magnetic bead-conjugated anti-CD102 antibodies (Biolegend). Organ culture In the organ culture experiments, 2 mm 2 tissue specimens were cultured in DMEM without or with FBS (2%) containing various stimulators for 5–6 h. All experiments were carried out in the presence of polymyxin B (10 μg ml −1 ). GST fusion proteins GST-fused constructs containing the murine SAA3 protein were generated in pGEX4T-1 (GE Healthcare). The proteins were expressed in Escherichia coli BL21 cells and purified on a glutathione-sepharose column. Protein purification from stable cell lines Mouse S100A8 and SAA3 genes with FLAG peptides at their carboxy termini were cloned into pcDNA5/FRT/TO-TOPO (Invitrogen). A stable cell line that displayed tetracycline-inducible expression of FLAG-tagged SAA3 was generated using the Flp-In system (Invitrogen) according to the manufacturer’s instructions. Immunohistochemistry To immunostain the frozen lung tissue sections, we used anti-mouse CCR2 (Santa Cruz), anti-CCL2 (R&D system), anti-mouse S100A8 (Santa Cruz), and rat anti-mouse MECA32 (BD Pharmingen) antibodies. For the paraffin-embedded human tissue sections, we used anti-CCR2 (Abcam), anti-fibrinogen (Dako), anti-A100A8 (BMA Biomedicals), and anti-S100A9 antibodies (BMA Biomedicals). We also used anti-mouse SAA3 antibody, as described previously [9] , and FITC-, Cy3- or Cy5-conjugated secondary antibodies were used to visualize the signals during confocal microscopy. The immunostained cell area values are shown as numbers of pixels normalized to the total surface area (1 × 10 6 pixels mm −2 , 0.3 mm 2 ). Immunoprecipitation and western blot analysis Lung tissues were lysed with lysis buffer (50 mM HEPES (pH 7.4), 1% Triton X-100, 150 mM sodium chloride, 1 mM ethylene glycol tetraacetic acid (EGTA) and 5 mM ethylenediaminetetraacetic acid (EDTA)) supplemented with protease inhibitor mixture, 1 mM phenylmethylsulfonyl fluoride, 1 mM sodium fluoride and 1 mM sodium orthovanadate. As shown in Fig. 4d , we used four antibodies for TLR4: (1) ab13556 (Abcam), (2) ab53629 (Abcam), (3) 558293 (BD Pharmingen) and (4) sc-12511 (Santa Cruz). For FAK detection, we used anti-pFAK (Tyr 397, Upstate) and anti-FAK (c-903, Santa Cruz) antibodies. Uncropped scans of the key western blots are provided in Supplementary Fig. S25 . Microarray analysis We re-analysed gene array data that were carried out previously (GEO accession code GSE5778 ) [8] . Quantitative-PCR Total RNA samples were isolated from frozen tissues using Trizol reagent (Invitrogen, Carlsbad, CA). Complementary DNA was synthesized with Superscript III reverse transcriptase and oligo dT primers (Invitrogen). Quantitative-PCR analysis was carried out using SYBR Green Master Mix, TaqMan Fast Advanced Master Mix (Applied Biosystems, CA), and the ABI 7500 Sequence Detection System. Gene expression levels were calculated from Ct values, and the relationship between the Ct value and the logarithm of the copy number of the target gene was confirmed to be linear using serial dilutions of the corresponding isolated DNA as a standard. In addition, gene expression levels were normalized to that of β-actin in each sample. The primer information was shown in Supplementary Methods . Statistical analysis All data are expressed as the mean±s.e.m. The Student’s t- test was used for all analyses. We considered P -values of <0.05 to be statistically significant. We used 8–10 mice (4–5 wild-type, 4–5 mutant mice) in each in vivo assay to obtain accurate phenotypes. In addition to our analyses of the experimental data, we also carried out analyses of small numbers of samples (N<5) using a non-parametric test (Mann–Whitney U -test). All of these latter tests produced statistically significant results ( P- value of <0.05), as was found with the Student’s t- test. How to cite this article: Hiratsuka, S. et al. Primary tumours modulate innate immune signalling to create pre-metastatic vascular hyperpermeability foci. Nat. Commun. 4:1853 doi: 10.1038/ncomms2856 (2013).